Transparent displays enabled by resonant nanoparticle scattering The ability to display graphics and texts on a transparent screen can enable many useful applications. Here we create a transparent display by projecting monochromatic images onto a transparent medium embedded with nanoparticles that selectively scatter light at the projected wavelength. We describe the optimal design of such nanoparticles, and experimentally demonstrate this concept with a blue-color transparent display made of silver nanoparticles in a polymer matrix. This approach has attractive features including simplicity, wide viewing angle, scalability to large sizes and low cost. Transparent display is a rapidly growing technology that enables many useful applications. With transparent displays, navigating information can be displayed on car windshields and aircraft cockpit windows; regular glass windows and even eyeglasses can become monitor screens for work or entertainment. A number of different transparent displays have been developed, each suitable for a subset of the applications. The simplest type is the head-up display that projects into the viewer's eyes through reflecting the image off a beam splitter [1] . Head-up displays are well suited to certain occasions, but the narrow viewing angle limits the position of the viewer. Diffusive screens achieve wider viewing angles by light scattering [2] ; such screens do not have wavelength selectivity, so stronger scattering is necessarily accompanied by lower transparency. Frequency-conversion screens achieve higher transparency using molecules that convert the projected ultraviolet light to visible light [3] , [4] , [5] , or infrared light to visible light [6] ; the conversion, however, is challenging to implement with high efficiency. Instead of relying on projection, one can also make electronic flat panel displays transparent, for example by combining organic light-emitting diodes with transparent electronics [7] , [8] , [9] . There is active research in developing this type of transparent displays, but scaling to large display sizes remains challenging. Given the limitations of these existing methods, it remains of great interest to explore new types of transparent displays. Here we create a transparent display by projecting monochromatic images onto a transparent medium embedded with nanoparticles that selectively scatter light at the projected wavelength. With the wavelength-selective scattering, such a screen can efficiently display the projected image while being highly transparent to the ambient light. After optimizing the design of such nanoparticles, we experimentally demonstrate this concept with a blue-color, broad viewing angle, transparent display made of silver nanoparticles in a polymer matrix. This method is simple, low cost and scalable to large sizes; these features make it attractive for some of the various transparent display applications. Concept Our approach is based on the fact that nanoparticles with sharp resonances can selectively scatter light of a particular wavelength, while being almost transparent at other wavelengths. By embedding wavelength-selective nanoparticles in a transparent medium and by projecting images at the resonant wavelength λ 0 , we can create a screen that scatters most of the projected light while being almost transparent to the broadband ambient light. This is illustrated in Fig. 1 . To implement a full-color display, one could use three types of nanoparticles, each selectively scattering light at one of the three desired colors: red, green and blue; alternatively, one could use a designed nanoparticle with multiple resonances, each lying at one of the three desired wavelengths. The challenge of a good implementation lies in making the resonances sharp while maintaining high transparency away from the resonances. 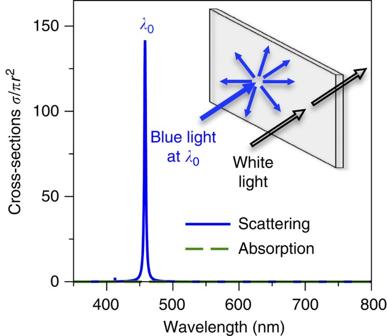Figure 1: Working principle for a transparent display based on wavelength-selective scattering from nanoparticles. The desired nanoparticles have the scattering cross-section sharply peaked at wavelengthλ0, and the absorption cross-section uniformly zero. A transparent medium embedded with such nanoparticles is transparent except for light at wavelengthλ0, as sketched in the inset. As an example, here we show the cross-sections for a metallic sphere in air, where the sphere has radiusr=15 nm, and the metal is described by the Drude model with plasma wavelength 260 nm and negligible dissipation; the absorption cross-section is negligible in this case. Figure 1: Working principle for a transparent display based on wavelength-selective scattering from nanoparticles. The desired nanoparticles have the scattering cross-section sharply peaked at wavelength λ 0 , and the absorption cross-section uniformly zero. A transparent medium embedded with such nanoparticles is transparent except for light at wavelength λ 0 , as sketched in the inset. As an example, here we show the cross-sections for a metallic sphere in air, where the sphere has radius r =15 nm, and the metal is described by the Drude model with plasma wavelength 260 nm and negligible dissipation; the absorption cross-section is negligible in this case. Full size image Theoretical design One way to achieve wavelength selectivity is using the localized surface plasmon resonances in metallic nanoparticles [10] , [11] , [12] , [13] , [14] . We first provide a rough estimate to determine which metal is optimal to use. For a small particle (particle size << wavelength) with dielectric function ∈ ( λ ), one can show that the ratio between on-resonance (at λ 0 ) and off-resonance (at λ 0 + Δ λ , for a small Δ λ of interest) scattering cross-sections is for particles of arbitrary shapes. The derivation is given in Methods. Equation (1) reveals that, for optimal wavelength-selective scattering, the desired material should have a small Im( ∈ ) and a fast-changing Re( ∈ ) near the resonance wavelength λ 0 . A metal with negligible loss would be ideal ( Fig. 1 provides one example; also see ref. Tribelsky and Luk'yanchuk), but most metals are quite lossy in the visible spectrum. 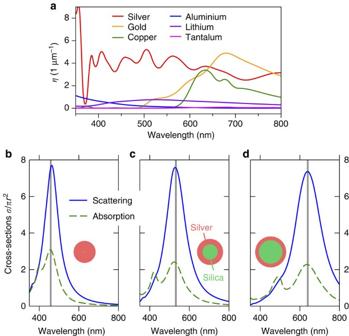Figure 2: Theory design for metallic nanoparticles suitable for displaying three different colors. (a) A performance estimator for the wavelength selectivity of small plasmonic particles. See text for the definition ofη. (b–d) Scattering and absorption cross-sections for silica-core silver-shell nanoparticles (embedded in ann=1.44 medium) optimized to scatter monochromatic light atλ0=458 nm (blue,b), 532 nm (green,c), and 640 nm (red,d). Insets show the relative sizes of the structures;ris the outer radius of the particle. Figure 2a shows the metals with large η ≡|R e ( d ∈ / dλ )/Im( ∈ )| 2 in the visible spectrum (refractive index from ref. Palik). Silver has the highest value of η for most of the visible spectrum, so we choose to work with silver-based nanoparticles. Figure 2: Theory design for metallic nanoparticles suitable for displaying three different colors. ( a ) A performance estimator for the wavelength selectivity of small plasmonic particles. See text for the definition of η . ( b – d ) Scattering and absorption cross-sections for silica-core silver-shell nanoparticles (embedded in an n =1.44 medium) optimized to scatter monochromatic light at λ 0 =458 nm (blue, b ), 532 nm (green, c ), and 640 nm (red, d ). Insets show the relative sizes of the structures; r is the outer radius of the particle. Full size image For more detailed optimization, we define a figure of merit (FOM) that captures the desired properties: a uniformly low absorption cross-section σ abs , a high scattering cross-section σ sca at λ 0 , and low σ sca elsewhere. The overline and the symbol max{…} denote the mean and the maximum in the visible spectrum (from 390 nm to 750 nm). The number 2 is a weighing factor chosen to balance sharp scattering and low absorption. The absolute value of the cross-section per particle is less important here because one can adjust the areal density of the nanoparticles on the screen; thus, the FOM is defined as a ratio. Also, in order to have a colorless transparent screen, we prefer a flat absorption spectrum, so we use max{ σ abs } rather than . One can also consider imposing a wavelength-dependent weight on the cross-sections to account for the spectral sensitivity of human eyes [15] , but we omit this weight for simplicity. With this FOM, we perform numerical optimizations on spherical core-shell nanoparticles with a silver shell and silica core, embedded in a transparent medium with refractive index n =1.44. Scattering and absorption cross-sections are calculated with the transfer matrix method [16] , using n =1.45 for silica and experimental values of the dielectric function for silver [17] . Particle size distribution is assumed to be a Gaussian with the standard deviation being 10% of the mean. We choose the core radius and shell thickness that maximize the FOM by performing a global optimization via the multi-level single-linkage algorithm [18] implemented within the free nonlinear optimization package NLopt [19] . The resonance wavelength λ 0 can be tuned to arbitrary colors. Figure 2b–d show the cross-sections of structures optimized to scatter monochromatic light at λ 0 =458 nm (blue), 532 nm (green), and 640 nm (red); the corresponding particle sizes and FOMs are listed in Table 1 . Table 1 Optimal particle sizes and FOM for silica-core silver-shell nanoparticles. Full size table According to the example in Fig. 1 , one would prefer σ sca to be even more narrow in wavelength; nevertheless, as we will see, one can obtain fairly good transparent display properties even with cross-sections comparable with those shown in Fig. 2 . Therefore, we leave it to future work to further improve the design. Dielectric nanoparticles may be a promising direction, as their resonance line widths are not as limited by absorption loss compared with metals [20] ; Supplementary Fig. 1 provides such examples. Utilizing higher-order resonances [21] , [22] , [23] , [24] is also a possible direction, provided that one can keep the lower-order broadband resonances out of the visible spectrum. The same FOM and optimization procedure can be applied in these explorations. Experimental realization As a proof of principle, we experimentally realize a blue-color-only transparent display. Simple spherical silver nanoparticles are used, since the structure optimized to scatter blue light has a negligible silica core ( Table 1 ). A transmission electron microscopy image of these particles (nanoComposix) is shown in the inset of Fig. 3a ; their diameter of 62±4 nm is chosen to match the optimized structure. To host the nanoparticles in a transparent polymer matrix, we mix 10% weight of polyvinyl alcohol (PVA, 80% hydrolyzed, Sigma-Aldrich) into an aqueous solution of silver nanoparticles (concentration 0.01 mg ml −1 ). We pour 480 ml of this liquid onto a framed square glass plate that is 25 cm in width, remove air bubbles from the liquid with a vacuum chamber and let the liquid dry out in the hood at room temperature. Over a course of 40 h, the liquid solidifies into a transparent polymer film of thickness 0.46 mm. This transparent thin film is the screen of our display. Its average transmittance is 60% in the visible spectrum (averaged from 390–750 nm). 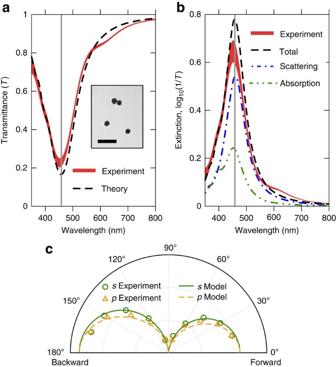Figure 3: Characterization of the fabricated film that is used as a transparent screen. (a) Transmittance spectrum of the film; width of the experimental curve indicates plus/minus one s.d. across different spots on the film. Inset shows a TEM image of the nanoparticles; the diameter is 62±4 nm. Scale bar, 200 nm. (b) Same data plotted as extinction, together with theory-predicted contributions from scattering and absorption. (c) Angular distribution of scattered light at 458 nm, when normally incident light has electric field polarized perpendicular (s) and parallel (p) to the scattering plane. The radial axis is in arbitrary units. Figure 3: Characterization of the fabricated film that is used as a transparent screen. ( a ) Transmittance spectrum of the film; width of the experimental curve indicates plus/minus one s.d. across different spots on the film. Inset shows a TEM image of the nanoparticles; the diameter is 62±4 nm. Scale bar, 200 nm. ( b ) Same data plotted as extinction, together with theory-predicted contributions from scattering and absorption. ( c ) Angular distribution of scattered light at 458 nm, when normally incident light has electric field polarized perpendicular ( s ) and parallel ( p ) to the scattering plane. The radial axis is in arbitrary units. Full size image Figure 3a shows the transmittance spectrum of this film. For a direct comparison with theory, the measured data are normalized by the transmittance of a plain PVA film of the same thickness (which is higher than 90% in the visible spectrum). Theory prediction (solid line in Fig. 3a ) from the calculated cross-sections and the Beer–Lambert law (no fitting variables) agrees well with the measured data; the slight discrepancy is due to a minor clustering of the nanoparticles ( Supplementary Fig. 2 ). The calculated cross-sections indicate that the on-resonance scattering is significantly stronger than the on-resonance absorption ( Fig. 3b ), which is good for our purpose here. Figure 3c shows the angular distribution of scattered light at λ 0 . The distribution is close to the Lambertian distribution for an ideal diffusely reflecting surface, confirming that the scattered light can be viewed from a wide angle. The polarization dependence is weak, indicating that we may operate the screen with incident light of arbitrary polarization. A minimal model for the angular dependence (described in Methods) yields the lines in Fig. 3c . In Fig. 4a , we show the transparent display at work, with a blue MIT logo projected onto the screen from a small laser projector (MicroVision SHOWWX+). This projector is suitable here since it functions by projecting monochromatic light from three laser diodes (red, green and blue) [25] ; we measure the wavelength of its blue light to be 458±2 nm. The projected image shows up clearly on our screen, and is visible from all directions. In comparison, the same image projected onto regular glass ( Fig. 4a , photo on the right) can barely be seen due to the lack of scattering. The transparency of our screen can be judged by comparing it with regular glass: Fig. 4a shows that objects behind the screen (three colored cups) remain visible, and their apparent color and brightness change only very slightly. A recording of the screen displaying animated images is shown in Supplementary Movie 1 . We also compare an image projected onto this screen and onto a piece of white paper: Fig. 4b shows that on our screen, the projected image is slightly dimmer but the contrast is better due to less scattering of ambient light. Finally, we point out that high-resolution images can be projected onto this screen with clarity, because the screen has on average 6 × 10 9 nanoparticles per cm 2 of area. 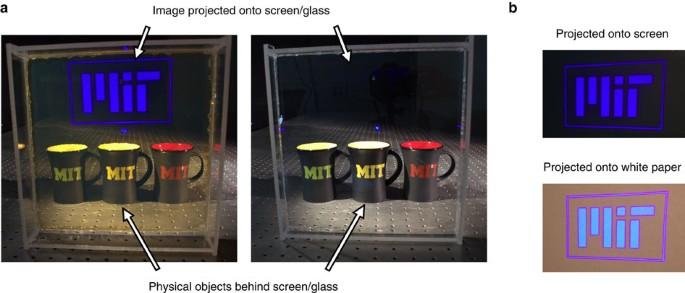Figure 4: Demonstration of a blue-color transparent display. (a) Photographs showing the transparent screen (left) in comparison with a regular piece of glass (right). A laser projector projects a blue MIT logo onto both the transparent screen and the regular glass; the logo shows up clearly on the transparent screen, but not on the regular glass. Three cups are placed behind to visually assess the transparency. (b) Photographs comparing letters projected onto the transparent screen (top) and onto a piece of white paper (bottom). In bothaandb, the pair of photographs are captured with the same lighting condition and exposure, and photographs are not edited. See alsoSupplementary Movie 1. Figure 4: Demonstration of a blue-color transparent display. ( a ) Photographs showing the transparent screen (left) in comparison with a regular piece of glass (right). A laser projector projects a blue MIT logo onto both the transparent screen and the regular glass; the logo shows up clearly on the transparent screen, but not on the regular glass. Three cups are placed behind to visually assess the transparency. ( b ) Photographs comparing letters projected onto the transparent screen (top) and onto a piece of white paper (bottom). In both a and b , the pair of photographs are captured with the same lighting condition and exposure, and photographs are not edited. See also Supplementary Movie 1 . Full size image We have proposed and demonstrated transparent displays enabled by the wavelength-selective scattering of nanoparticles. Decent transparency and scattering efficiency have been achieved with our proof-of-concept demonstration, and this method has additional attractive features including simplicity, wide viewing angle and scalability to large sizes. The method is also economical: in our experiment, the polymer is inexpensive, and only 7 μg of silver nanoparticles is used per cm 2 of screen. The natural next step of this method will be achieving narrower line-width for the scattering while maintaining transparency away from the resonance; this will further enhance transparency, and will be important for the realization of a full-color transparent display. Finally, we point out a few extensions of this transparent display method. First, with a flexible polymer matrix, we can potentially realize flexible and scrollable transparent displays. Second, since most light undergoes single scattering (the thickness of the film, 0.46 mm, is comparable to the mean free path at resonance, 0.26 mm) instead of multiple scattering, the scattered light retains the polarization of the incident light. Therefore, one can achieve three-dimensional viewing effect by projecting two images simultaneously (one right-handed circularly polarized and one left-handed circularly polarized) and viewing the superimposed image with polarized glasses. Third, by placing a black cloth behind such a transparent screen, one can also create a black screen (non-transparent) that has higher contrast than a traditional white screen: as shown in Fig. 4b , a traditional white screen may have low contrast due to the diffuse scattering of ambient light, but the transparent screen does not. Resonant scattering of small plasmonic particles For a particle much smaller than the wavelength λ of the incident light, the local electromagnetic field has almost no spatial variation. We can calculate the optical response from such a particle using the quasi-static approximation (also called dipole approximation) [26] . Here we apply this method to estimate the sharpness of the scattering cross-section for small plasmonic particles of arbitrary shapes. In the quasi-static approximation, the scattering cross-section σ sca averaged over angle and polarization of the incoming light is [26] where is the wavenumber in the surrounding medium, and α 1,2,3 are the static electric polarizabilities of the particle in three orthogonal polarizations. Localized surface plasmon resonances occur at the wavelength λ 0 for which For a sphere, this condition simplifies to Re( ∈ ( λ 0 )) =−2 ∈ m ; here we work with the more general expression that is applicable to arbitrary shapes. We denote the real and imaginary parts of the on-resonance (at λ 0 ) and off-resonance (at λ 0 + Δ λ , for a small Δ λ of interest) dielectric constants as assuming and . We write the polarizability as a rational function, α j ( ∈ )= N ( ∈ )/ D ( ∈ ), and let the polynomial in the denominator be D ( ∈ ) = ∑ n =0 c n ∈ n . Using the fact that D ( ∈ r )=0, we can subtract D ( ∈ r ) from the off-resonance D ( ∈ ), and take out the common factor to get only the first square bracket is of interest to us, since none of the terms in the second square bracket depends on Δ λ . With this observation, we see that the ratio between on-resonance and off-resonance scattering cross-sections is approximately which proves equation (1). With this result, we can estimate the sharpness of the scattering cross-section using only the dielectric function ∈ ( λ ) of the metal. However, we note that the resonance condition, equation (4), requires materials with negative Re( ∈ ), so this result can only be applied to plasmonic resonances. Angular distribution model The overall trend of the angular distribution can be described by a factor f 1 =cos θ that accounts for the observed area at angle θ ; this is the Lambertian distribution. To account for the polarization dependence, we consider a single-scattering event from a small particle, which has a factor and for electric field polarized perpendicular or parallel to the scattering plane [26] ; here θ′ is the angle inside the PVA film, given by , where n =1.44 is the refractive index of PVA. We also account for the transmission coefficient f 3 from PVA to air, given by Fresnel equations. Finally, light scattered to the back side is attenuated by absorption, which we estimate to be around 20%, so we include an additional factor of f 4 =0.8 for θ <90 deg., f 4 =1 for θ > 90 deg. Combining these factors, we model the angular dependence as f 1 f 2 f 3 f 4 . Prediction of this minimal model is plotted in Fig. 3c . How to cite this article : Hsu, C. W. et al. Transparent displays enabled by resonant nanoparticle scattering. Nat. Commun. 5:3152 doi: 10.1038/ncomms4152 (2014).